Imaging single cells in a beam of live cyanobacteria with an X-ray laser There exists a conspicuous gap of knowledge about the organization of life at mesoscopic levels. Ultra-fast coherent diffractive imaging with X-ray free-electron lasers can probe structures at the relevant length scales and may reach sub-nanometer resolution on micron-sized living cells. Here we show that we can introduce a beam of aerosolised cyanobacteria into the focus of the Linac Coherent Light Source and record diffraction patterns from individual living cells at very low noise levels and at high hit ratios. We obtain two-dimensional projection images directly from the diffraction patterns, and present the results as synthetic X-ray Nomarski images calculated from the complex-valued reconstructions. We further demonstrate that it is possible to record diffraction data to nanometer resolution on live cells with X-ray lasers. Extension to sub-nanometer resolution is within reach, although improvements in pulse parameters and X-ray area detectors will be necessary to unlock this potential. Imaging live cells at a resolution higher than the resolution of optical microscopy is a significant challenge. Fluorescence microscopy can achieve a degree of super-resolution via labelling cellular components with a dye, but only on the labelled regions of the cell [1] . Achieving nanometer or sub-nanometer resolution would require high-energy radiation with shorter wavelength than optical light. X-rays and electrons have the requisite wavelengths and would be suitable for such studies; however, these probes also cause significant radiation damage. A dose in excess of 100,000,000 Gray (Gy, J kg −1 ) would be required to reach nanometer resolution on a cell, and no cell can survive this. A dose of 20 Gy causes certain death in humans, 60–800 Gy kills most cells, and 25,000 Gy is lethal to all known organisms [2] , [3] . As a consequence, much of what we know about cells at high resolution comes from dead material. Theory predicts [4] that an ultra-short and extremely bright coherent X-ray pulse from an X-ray laser can outrun key damage processes to deliver a molecular-level snapshot of a large macromolecule, a virus, or a cell [5] that is alive at the time of image formation [5] . This principle of ‘diffraction before destruction’ exploits the difference between the speed of light (the X-ray pulse) and the much slower speed of damage formation. The femtosecond pulse ‘freezes’ motion at physiological temperatures on the time scale of atomic vibrations, offering unprecedented time resolution [6] . Conventional experiments performed at synchrotrons [7] , [8] , [9] , [10] used cells that were either fixed and frozen, or dried, and these cells were not alive. Other studies use wet cells that were alive at the start of the exposure but were then killed by the first millionth of the X-ray dose needed to obtain the diffraction pattern [11] . Flash diffractive imaging overcomes these problems. We first demonstrate that live cyanobacteria can be efficiently aerosolized, and a beam of live cells can be introduced into the pulse train of an X-ray laser at low pressure. We then show that we can record high-quality diffraction patterns on such cells with practically no scattered background. We retrieve phases directly from the diffraction patterns to reconstruct images, using a variant [12] of the Gerchberg-Saxton-Fienup phase retrieval algorithm [13] , [14] , and present the reconstructed exit-wavefronts as synthetic X-ray Nomarski images [15] . These images are similar to what one would expect to see with differential contrast microscopy, only at the higher resolutions available using X-rays. Finally, we present experimental evidence that diffraction data to nanometer resolution can be recorded on live cells using our method of ‘diffraction before destruction’. Live cells Cyanobium gracile and Synechococcus elongatus cells were selected for these studies because of their small size, robustness and convenient autofluorescence properties that can be used to assess cell viability [16] . Cyanobacteria are tough and can be found in hot and cold environments, including volcanic regions and the polar ice caps. Solitary C. gracile and S. elongatus cells have an oval-to-cylindrical shape, and vary in size between 0.25–0.4 μm in diameter and 0.4–4.0 μm in length [17] . Cell division occurs symmetrically by binary fission. The two daughter cells separate from each other after reaching the size and shape of the mother cell [18] . We used non-synchronized cell cultures undergoing active growth to provide cells in various stages of their cell cycle. Injected cells arrive in random order and are imaged in random orientations. Aerosol sample injection Aerosol injection [19] , [20] delivers samples without interference from any container or substrate and is capable of producing millions of shots per day for high-throughput studies at very low noise levels. Other methods employ membranes [21] or closed containers [22] . Everything that is illuminated by a pulse of an X-ray laser is ‘sample’ in coherent diffractive imaging, including the structure of the sample holder, the liquid column of a liquid jet or materials that make up microfluidic devices. Such sample holders contribute to scattering and increase unwanted noise. Aerosol injection removes this clutter and assures that the sample is clearly isolated from its surroundings, and this is important for phasing. Aerosols play various roles in biology. A large number of infectious diseases are transmitted via aerosols. Ocean sprays put out about 3.5 × 10 12 kg aerosol per year from jet drops formed when bubbles burst on wave crests [23] and can carry live cells (like those studied here) over wide areas. Aerosols are also widely used in scientific and medical applications. A recent study shows that bio-electrosprayed multicellular zebrafish embryos are viable and develop normally [24] . Cell sorters use microdroplets to separate different cells from each other. Similarly, the new science of tissue printing [25] , [26] is based on the use of microdroplets to deliver cells to pre-defined positions. We exploit similar processes in this study to bring living cells into the gas phase for a brief period of time and to deliver these cells into the pulse train of the Linac Coherent Light Source (LCLS) as a narrow beam ( Fig. 1 ). 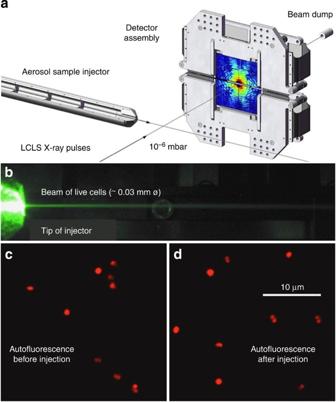Figure 1: The experimental arrangement. (a)C. gracilecells were injected into the pulse train of the LCLS36at 10−6mbar pressure, using an aerosol sample injector built in Uppsala. The direct beam passes through an opening in the centre of the two detector halves37. (b) Photograph of the beam of live cyanobacteria exiting the injector and illuminated by a green laser beam. (c,d) Fluorescence micrographs ofC. gracilecells before (c) and after (d) injection indicate the cells remained intact. Injected cells were captured on a microscope slide in front of the injector, and the slide was transferred to atmospheric pressure to record the micrograph in (d). Figure 1: The experimental arrangement. ( a ) C. gracile cells were injected into the pulse train of the LCLS [36] at 10 −6 mbar pressure, using an aerosol sample injector built in Uppsala. The direct beam passes through an opening in the centre of the two detector halves [37] . ( b ) Photograph of the beam of live cyanobacteria exiting the injector and illuminated by a green laser beam. ( c , d ) Fluorescence micrographs of C. gracile cells before ( c ) and after ( d ) injection indicate the cells remained intact. Injected cells were captured on a microscope slide in front of the injector, and the slide was transferred to atmospheric pressure to record the micrograph in ( d ). Full size image Cells were transferred into a volatile buffer before aerosolisation to avoid formation of surface deposits during the evaporation of microdroplets. A variety of volatile buffers can be used to maintain pH and to provide suitable osmotic conditions. Here we used 25 mM ammonium acetate at pH 7.5. By adjusting temperature, humidity and gas flow, the amount of water on the sample can be controlled. The suspension of live cells was aerosolized with a gas-dynamic virtual nozzle [27] with helium. In the nozzle, a converging stream of pressurised helium squeezes a 20 μm wide liquid column into a 1 μm jet. The reduction of diameter leads to fluid acceleration, and the liquid column accelerates from 0.06 m s −1 (the velocity of the liquid in the 20 μm column) to about 100 m s −1 (in the 1 μm jet) in a distance of about 100 μm. Inside this short acceleration zone, the fluid is moving 1 m s −1 faster at the front of a 1 μm object than at the back of it. This occurs for a brief period (~2 microseconds) after which the jet continues as a plug flow. In contrast to fixed-diameter nozzles, the orifice of the gas-dynamic nozzle is ‘flexible’ and lets larger clumps pass. Cells are highly elastic (elastic modulus 0.2–100 kPa [28] ) and are in fact orders of magnitude more elastic than a latex condom whose elastic modulus is ~2 MPa [29] . As a result, cells respond elastically to a broad range of shear conditions [30] . Some distance away from the constriction zone, the 1 μm jet breaks into droplets in a spontaneous process governed by surface tension. Controlled evaporation of the aerosol droplets cools the sample, and the adiabatically cooled aerosol is then guided through an aerodynamic lens to produce a narrow beam of living cells as shown in Fig. 1b . Femtosecond serial nanocrystallography [31] uses these nozzles to introduce sensitive protein crystals into the X-ray beam. The difference is that we shoot our samples after the jet breaks into droplets and the buffer has evaporated while nanocrystallographers shoot their samples inside the jet itself. Figure 1c,d shows that this type of sample injection is not disruptive, and the shape and the autofluorescence of the injected cells remain unchanged. This is not quite unexpected. Aerosols of cyanobacteria can be carried for long distances, and metabolically active cells have been detected at altitudes of 20–70 km where atmospheric pressure drops to below a millibar [32] , [33] , [34] . We also tested the survival of E. coli cells by capturing and culturing injected cells (F.N.A., unpublished). The results show that E. coli cells survive the process of sample injection. One of us (R.K.) injected brewers yeast, collected it and subsequently demonstrated anaerobic metabolism and growth (R.K. unpublished). Nevertheless, not all sample types may be amenable to aerosol sample injection, and cell lines should be tested before experiments. There is room for other methods, for example, using the jet itself, as in nanocrystallography, for experiments where buffer exchange is not possible (but the excess liquid of the jet will contribute to scattering). Our aim is to attempt very high-resolution studies on small living cells, and this requires small and truly isolated cells without excess scattering material. Data collection Experiments were carried out at the Atomic, Molecular and Optics (AMO) end-station [35] of the LCLS [36] at 517 eV (2.40 nm wavelength) and at 1,100 eV (1.13 nm) photon energy. The length of the photon bunch (full-duration at half-maximum) was about 70 fs (see Methods). The pulse was focused to a spot of 3 μm × 7 μm (full width at half maximum). The average photon density in the focus was about 1.1 × 10 11 photons per pulse μm 2 at 517 eV, and 8.6 × 10 10 photons per pulse μm 2 at 1,100 eV. Far-field diffraction patterns were recorded on a pair of pnCCD detectors [37] in the CFEL-ASG Multi Purpose (CAMP) instrument [37] . The detectors were read out at the 120 Hz repetition rate of the LCLS. We used the Condor software package ( http://www.github.com/mhantke/condor ) to optimize experimental conditions. We collected diffraction patterns of C. gracile cells for 60 min at a hit ratio of 43% and selected the 7,500 clear single hits for further analysis, using the Cheetah software package [38] . The diffraction pattern of a non-crystalline object is continuous, and phases can be recovered directly from such patterns [39] , [40] , [41] , using an iterative process [12] , [13] , [14] . We used the Hawk software package [42] for phasing (Methods). Successful phase retrieval requires accurately measured low-resolution data. This is not a trivial problem because strong hits saturate the detectors at low diffraction angles. As a compromise, we selected medium-strong hits, which contained either no, or only a few saturated pixels, while still providing data to reasonably high resolution ( Fig. 2a–j , Methods). These patterns were analysed for weakly constrained modes, using methods described in ref. 19 . The analysis revealed no unconstrained modes in the reconstructions. 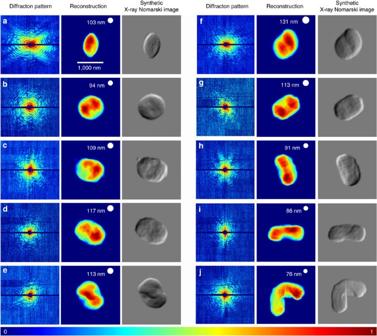Figure 2: Diffraction patterns and reconstructed electron densities for liveC. gracilecells. The cells were alive when the femtosecond pulse traversed them but exploded some picoseconds later5,52. Photon energy: 517 eV (water window), sample-to-detector distance: 740 mm. The total number of scattered photons in the diffractions patterns varies between 0.5 and 5 million. Each reconstructed image is the average of up to 400 independent reconstructions (Methods). Resolution was estimated from the phase retrieval transfer function as described in Methods. White circles in the reconstructions indicate the resolution relative to the object size. Features smaller than the circles need to be interpreted with care. Reconstructions are normalized to a 0-1 scale (colour bar) and are sorted according to cell size. Synthetic X-ray Nomarski images were calculated from the complex-valued reconstructions15to show the reconstructed phase shift properties of the object together with its density. Figure 2: Diffraction patterns and reconstructed electron densities for live C. gracile cells. The cells were alive when the femtosecond pulse traversed them but exploded some picoseconds later [5] , [52] . Photon energy: 517 eV (water window), sample-to-detector distance: 740 mm. The total number of scattered photons in the diffractions patterns varies between 0.5 and 5 million. Each reconstructed image is the average of up to 400 independent reconstructions (Methods). Resolution was estimated from the phase retrieval transfer function as described in Methods. White circles in the reconstructions indicate the resolution relative to the object size. Features smaller than the circles need to be interpreted with care. Reconstructions are normalized to a 0-1 scale (colour bar) and are sorted according to cell size. Synthetic X-ray Nomarski images were calculated from the complex-valued reconstructions [15] to show the reconstructed phase shift properties of the object together with its density. Full size image Image reconstruction Figure 2a–j shows the reconstructed exit-wavefronts (images) for 10 live C. gracile cells together with the corresponding diffraction patterns. The reconstructions represent two-dimensional (2D) projections of the electron density of the cells. The images are arranged by increasing size and show the expected morphologies of cells during division [17] , [18] . For the sake of comparison, Fig. 3a–i shows live C. gracile cells imaged by conventional Nomarski differential interference contrast microscopy in an optical microscope. 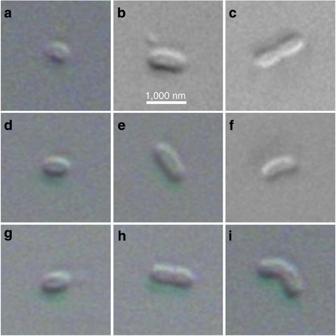Figure 3: Optical Nomarski images of LiveC. gracilecells. Panelsa–ishow images of liveC. gracilecells imaged at an optical microscope equipped with differential contrast Nomarski optics. Figure 3: Optical Nomarski images of Live C. gracile cells. Panels a – i show images of live C. gracile cells imaged at an optical microscope equipped with differential contrast Nomarski optics. Full size image Each reconstruction in Fig. 2 was repeated 400 times, starting from different and independent random phases. We used hierarchical clustering and an analysis of Fourier-errors and real-space errors to assess the quality of reconstructions (Methods). We also calculated synthetic X-ray Nomarski differential interference contrast images [15] from the complex-valued reconstructions to present the reconstructed cells in a familiar form. These X-ray Nomarski images have the same spatial resolution as the reconstructions in Fig. 2 , but display the object in a similar manner to what one would expect to see in a Nomarski microscope at room temperature, only at a higher resolution available using X-rays. We use the phase retrieval transfer function (PRTF) [43] to assess the resolution of the reconstructions, and define resolution according to where the PRTF drops below 1/ e (Methods, refs 19 , 44 ). The diffraction patterns contain data to higher resolution than the resolution of the reconstructions indicated on Fig. 2 (the full-period resolution at the edge of the detector was 46 nm and 33 nm in the corner at 517 eV). The results presented here show we can successfully introduce living cells into the beam of the LCLS without a container, hit them at high hit rate and reconstruct the exit-wavefront from the low-noise data. Detector saturation limited the achievable resolution. In fact, the reconstructions shown in Fig. 2 come from relatively weak exposures that did not saturate the detectors (Methods). A number of much stronger exposures were also recorded, and in some of these exposures the diffraction signal extended to nanometer resolution. 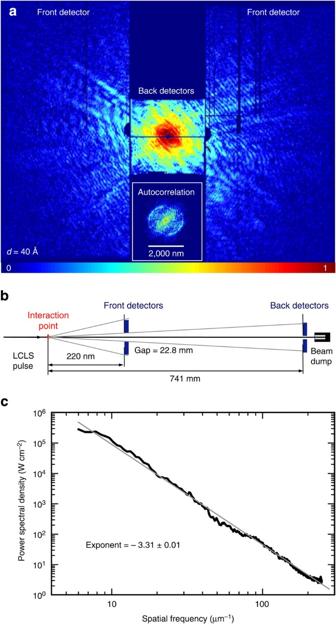Figure 4: Data extend to 4 nm full-period resolution in a strong exposure. (a) Diffraction pattern of a micron-sizedS. elongatuscell at 1,100 eV photon energy (1.13 nm wavelength) with ~1011photons μm−2on the sample in ~70 fs. The size of a small protein molecule is 4 nm. The signal to noise ratio at 4 nm resolution was 3.7 with 0.24 photons per Nyquist pixel. The cell was alive at the time of the exposure. The central region of the pattern (dark red) is saturated and this prevented reliable image reconstruction. The pnCCDs saturate at 1,330 photons per pixel at 1,100 eV photon energy. (b) Arrangement of four pnCCD detectors for high-resolution imaging. Each pnCCD had 1,024 × 512 pixels and an active area of 76.8 mm × 38.4 mm. (c) Signal decline with spatial frequency. The vertical scale is based on azimuthally averaged photon numbers per pixel area and corresponds to the power density in the pattern over the 70 fs exposure. The exponent of the signal decay (−3.31±0.01) matches simulations45. Figure 4 shows one such pattern for a live S. elongatus cell at 1,100 eV photon energy, 70 fs pulse length, about 10 11 photons μm −2 on the sample. Four pnCCD detectors were used to record this pattern ( Fig. 4b ). The central back detector in Fig. 4 is identical to the detector used in Fig. 2 . In this strong hit, a large part of the back detector was saturated (dark red in Fig. 4a ), preventing reliable phasing, but the signal extended to 4 nm resolution on the front detectors, which is the size of a small protein molecule. More than 58 million scattered photons were recorded on the back detectors, and 1.3 million on the front detectors. The size of the cell was derived from the autocorrelation. Figure 4c shows that in a log/log representation the drop-off of the signal is linear with spatial frequency in the range covered by our measurements, and the exponent of the signal decay is −3.31±0.01, matching simulations [45] . Figure 4: Data extend to 4 nm full-period resolution in a strong exposure. ( a ) Diffraction pattern of a micron-sized S. elongatus cell at 1,100 eV photon energy (1.13 nm wavelength) with ~10 11 photons μm −2 on the sample in ~70 fs. The size of a small protein molecule is 4 nm. The signal to noise ratio at 4 nm resolution was 3.7 with 0.24 photons per Nyquist pixel. The cell was alive at the time of the exposure. The central region of the pattern (dark red) is saturated and this prevented reliable image reconstruction. The pnCCDs saturate at 1,330 photons per pixel at 1,100 eV photon energy. ( b ) Arrangement of four pnCCD detectors for high-resolution imaging. Each pnCCD had 1,024 × 512 pixels and an active area of 76.8 mm × 38.4 mm. ( c ) Signal decline with spatial frequency. The vertical scale is based on azimuthally averaged photon numbers per pixel area and corresponds to the power density in the pattern over the 70 fs exposure. The exponent of the signal decay (−3.31±0.01) matches simulations [45] . Full size image In synchrotron X-ray microscopy, the maximal attainable resolution on non-living biological particles is limited to about ~10 nm (ref. 46 ). Unfortunately, synchrotron radiation kills live cells long before any measurable signal can be accumulated, and, as a consequence, no living cell has ever been imaged at any reasonable resolution at a synchrotron (cells were dried, frozen and so on). ‘Diffraction before destruction’ overcomes this problem and can give high-resolution data, but it only permits one shot from the sample, corresponding to a spherical section through the Fourier amplitudes of the object. Three-dimensional structure determination is possible for identical objects exposed to the beam one-by-one in different orientations; this however cannot be done easily with non-identical objects, such as cells (for a survey, see ref. 2 ). Methods have been proposed for the simultaneous illumination of cells from multiple directions to provide a 3D view of the object [5] , and instrumentation to achieve this is under development. Although 3D imaging would be highly desirable, studies on living cells are based almost entirely on 2D images. Clinical and research laboratories around the world utilize 2D projections of cells. The cells are usually not labelled, and their features are brought out by phase-contrast techniques in a similar manner as in our present study. Specific labelling techniques are available for X-ray diffraction microscopy and can be used for the selective identification of components [47] . According to predictions [5] , data to sub-nanometer resolution may be recorded on micron-sized living cells through ‘diffraction-before-destruction’ [4] . Physical limits to resolution in the pattern are related to sample size and composition, pulse duration, pulse intensity, wavelength and the movement of the sample during exposure [5] . No fundamental limit has been encountered so far with pulses presently available from the LCLS, and the results presented here are in agreement with predictions [4] , [5] , [45] . It is, however, not trivial to image large objects, like small living cells, at high resolution. In evaluating resolution we make a distinction between resolution in the signal and in the reconstruction. We have recorded data beyond 4 nm resolution, and reconstructed images up to a resolution of 76 nm. These are still the highest resolution recordings and reconstructions of living cells using coherent diffractive imaging. To reach nanometer resolution in reconstructions, we need to meet the following requirements. The diffraction signal fades away with an exponent of −3.31 over the range of spatial frequencies probed in our measurements ( Fig. 4c ). Accurate measurement of nanometer signal requires very low background. Container-free sample injection delivers truly isolated samples into the X-ray beam to record diffraction patterns with low scattered background. Under these conditions, signal from the sample can be measured to the highest possible resolution over a flat background. The contrast between the sample and its surrounding (wet helium gas expanding into a vacuum chamber pumped to 10 −6 mbar) is high. The clean background and the high contrast are important for the finite support constraint in phase retrieval. We estimate that nanometer resolution in the signal of a micron-sized cell would require a pulse with duration shorter than 10 fs and around 10 12 –10 13 photons μm −2 on the sample [5] at 3–10 keV photon energy. Resolution in a 2D reconstruction from a single exposure depends on the success of phase retrieval, and is also influenced by the lift-off of the Ewald sphere from the projection plane at high angles (shorter wavelengths would alleviate this problem). The projection approximation also presumes that the Born approximation is valid. This requires harder X-rays for samples thicker than those studied here. The maximal size of an object for successful reconstruction is currently limited to about 1-2 μm at the LCLS for a number of reasons. First, the bandwidth of an LCLS pulse is ~0.2% and this gives about 500 resolution elements in an image. If a target resolution of 2 nm is aimed for, the object size cannot be bigger than about 1 μm. Smaller bandwidth would allow studies on larger objects. An oversampled diffraction pattern is necessary for phase retrieval [48] . Second, the focus must be large enough to cover the sample yet contain enough photons to produce strong scattered signal from the cell. A larger focus requires more photons per pulse and these extra photons are currently not available from the LCLS. This limits the maximal useful focus size, which in turn limits the object size to about 1-2 μm. Missing low-resolution data pose perhaps the largest problem in image reconstruction. Low-resolution terms are crucial for the determination of the support for the object. The X-ray detector has a hole at its centre to let the direct beam pass through. The size of this blind spot limits the maximal object size to 1-2 μm at the relevant wavelengths. In strong exposures, there is a further and significant loss of low-resolution data due to detector saturation as can be seen in Fig. 4a . No fundamental limit has been encountered so far. The current limitations are technical. A femtosecond exposure ‘freezes’ all cellular processes at room temperature, including diffusion, and thus eliminates blurring. This is an advantage over other cell-imaging methods and will become important if or when nanometer resolution will be achieved on a micron-sized cell. Stronger and shorter pulses, like those expected from the European XFEL ( www-library.desy.de/preparch/desy/2011/desy11-152.pdf ) could bring high-resolution cellular imaging within reach. Experimental set-up The experiment was executed using the CFEL-ASG Multi-Purpose (CAMP) instrument [37] , at the AMO end station [35] of the LCLS [36] . The photon energy was 517 eV (2.40 nm wavelength) for Fig. 2a–j ,1,100 eV (1.13 nm) for Fig. 4a . The bandwidth of the LCLS is about 0.5%. The length of the electron bunch was 70 fs (full-duration at half-maximum, FDHM) but the length of the photon bunch is believed to be shorter. The photon bunch contained ~1.5 × 10 13 photons (1.26 mJ) at 517 eV, and 1.2 × 10 13 photons (2.14 mJ) at 1,100 eV. Only about 15% of the photons made it through the optics of the beam line, giving an average of about 1.1 × 10 11 photons μm −2 in the focus at 517 eV, and 8.6 × 10 10 photons μm −2 at 1,100 eV. The size of the focal spot was 3 μm × 7 μm (full-width at half-maximum). The CAMP chamber was equipped with two pairs of pnCCD [37] X-ray area detectors (front and back detectors), each consisting of two movable detector panels. The front detector assembly was placed 220 mm from the interaction point, and the back detector assembly at 741 mm. The direct beam exited through an opening between the two detector halves and was absorbed in a beam dump behind the detectors. Each detector panel contained 512 × 1024 pixels with 75 μm edge lengths and a full-well capacity of 500,000 electrons per pixel, corresponding to 2,833 photons at 517 eV (2.40 nm) and 1,333 photons at 1,100 eV (1.13). The read-out rate matched the 120 Hz repetition rate of the LCLS. Cells Cyanobium gracile PCC 6307 and Synechococcus elongatus PCC 7942 cells were grown in Bg11 medium in batch cultures under constant light. Before the imaging experiments, cells were centrifuged at 6,500 g for 10 min to create a soft pellet. The pellet was re-suspended in 25 mM ammonium acetate, and the buffer exchange was repeated twice to remove salt and contaminants. Optical microscopy We used a Zeiss AxioImager A1 fluorescence microscope equipped with Nomarski optics and a Zeiss Colibri laser source. Sample injection The suspension of live cells was aerosolized with helium in a gas dynamic nebulizer [27] , and delivered into the pulse train of the LCLS through an aerodynamic lens, using methods developed for our studies on giant viruses [19] . This method delivers cells without a container, minimizes background scattering and can produce millions of shots per day for high-throughput studies. Most of the nebulizing gas and vapours of the volatile buffer were pumped away through a differential pumping stage, and the concentrated and adiabatically cooled aerosol of cells was guided through an aerodynamic lens in a wet helium atmosphere, forming a narrow beam of live cells inside the vacuum chamber. The sample consumption was 2–4 μl min −1 from a solution of 10 11 cells ml −1 . The pressure inside the chamber was 10 −6 mbar. Data preprocessing The stream of raw data was monitored with the CASS [49] software during data collection. Subsequent processing of the raw data included background subtraction, masking of faulty pixels and correction for non-linear detector response, a task performed by the Cheetah software package [38] . Electronic noise was removed by subtracting the average value of 1,000 dark exposures. Bad pixels, over saturated pixels and insensitive pixels were masked out. The original patterns were down-sampled two-by-two for the reconstructions. Hit finding Hits were identified with the Cheetah software package [38] ( http://www.desy.de/~barty/cheetah ). Data were collected for 60 min, at a hit ratio of 43%, and we selected the 7,500 strongest hits from the exposures for further analysis. Hundred ‘weak’ patterns were then manually selected on having the least saturation, the right object dimensions and signals extending to reasonably high resolution. Reconstruction Phases were retrieved with the Hawk software package [42] . For each pattern, 400 reconstructions were made, starting from random initial phases. These reconstructions consisted of 5,000 iterations with the RAAR algorithm [12] , using a Shrinkwrap algorithm [50] for support determination, and concluded with 100 iterations by the ER algorithm [13] . No additional constraints such as enforcing the object to be real-valued were used, as we anticipate the effects of absorption in the thick cells to give effects similar to a phase object. We appreciate the fact that advanced phase retrieval algorithms such as RAAR [12] and HIO [14] are not designed to descend into the lowest point in the minimum, instead they strike a balance between the ability to identify minima and the ability to escape from shallow and presumably non-ideal minima. Therefore, we always finish the phase retrieval process with a number of iterations of ER [13] , which is known to guide the solution towards the lowest point of the minimum where the iterate currently resides. In our case we used 100 iterations for the ER refinement. We found that the ER refinement decreased the Fourier-error [50] by a factor of 14 on average and also improved the resolution to about two-thirds compared with solutions without ER refinement. Resolution for the reconstructions was estimated from the PRTF ( Fig. 5a–j ). The PRTF represents the confidence with which the diffraction phases have been retrieved. Many independent reconstructions are needed from each diffraction pattern to calculate the PRTF. The PRTF is equal to one when phases are consistently retrieved and zero when the phases are unknown. We define the resolution of the reconstructed images according to where the PRTF drops to 1/ e (refs 21 , 44 ). This is an arbitrary limit. 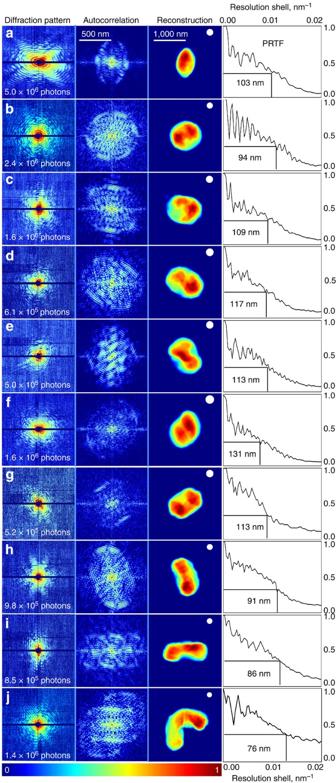Figure 5: Data quality and image resolution for liveC. gracilecells. (a–j) For each reconstruction, the diffraction pattern, the filtered autocorrelation function, and the reconstructed electron density together with the corresponding phase-retrieval transfer function (PRTF). The number of scattered photons in the patterns varied between 0.5 and 5 million. To mitigate distortion in the autocorrelation due to missing low-resolution data, we applied a filter introduced in ref.43. All images were normalized to a 0–1 scale, indicated by the colour bar. The white circles in the reconstructions indicate the resolution relative to the object size. Figure 5: Data quality and image resolution for live C. gracile cells. ( a – j ) For each reconstruction, the diffraction pattern, the filtered autocorrelation function, and the reconstructed electron density together with the corresponding phase-retrieval transfer function (PRTF). The number of scattered photons in the patterns varied between 0.5 and 5 million. To mitigate distortion in the autocorrelation due to missing low-resolution data, we applied a filter introduced in ref. 43 . All images were normalized to a 0–1 scale, indicated by the colour bar. The white circles in the reconstructions indicate the resolution relative to the object size. Full size image Each reconstruction was repeated 400 times with independent and random starting phases. The standard method to remove outliers among the reconstructions involves applying a threshold to the Fourier error before calculating a PRTF and averaging the images. We did, however, observe that qualitatively very different reconstructions could have very similar Fourier- and real-space errors ( Fig. 6a–f ). There is therefore a need for a more advanced method to identify outliers, than those currently used. We present here a method based on the clustering of reconstructions with the goal to both evaluate the standard method based on Fourier- and real-space error thresholds and to get a more reliable set of reconstructions from the measurements. 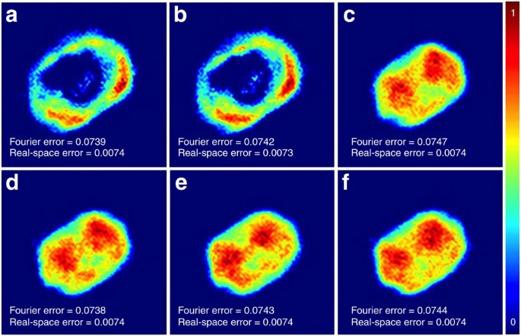Figure 6: Variance between reconstructions with similar Fourier and real-space errors. Six examples of individual reconstructions are shown, which have similar real-space and Fourier errors. (a,b) The only two outliers from 400 reconstructions starting from random phases. (c–f) Four of 398 very similar reconstructions. All images come from 400 individual reconstructions performed from pattern 7 ofFig. 5. The electron density was normalized to a 0–1 scale, indicated by the colour bar. Figure 6: Variance between reconstructions with similar Fourier and real-space errors. Six examples of individual reconstructions are shown, which have similar real-space and Fourier errors. ( a , b ) The only two outliers from 400 reconstructions starting from random phases. ( c – f ) Four of 398 very similar reconstructions. All images come from 400 individual reconstructions performed from pattern 7 of Fig. 5 . The electron density was normalized to a 0–1 scale, indicated by the colour bar. Full size image Selection of reconstructions We used hierarchical clustering and an analysis of Fourier-errors and real-space errors to assess the quality of reconstructions ( Figs 6 , 7 , 8 ). The UPGMA (Unweighted Pair Group Method with Arithmetic Mean) [51] hierarchical clustering algorithm was used to identify reproducible reconstructions ( Figs 7a–j and 8 ). The similarity function is the normalized scalar product between the reconstructions after translating them to their optimal fit. We plot the similarity in each cluster as a function of the number of clusters ( Fig. 7a–j ) and choose the agglomeration step where the plot makes a ‘kink’. This is a standard way to estimate the number of clusters and this capability is a reason for using this particular clustering algorithm. 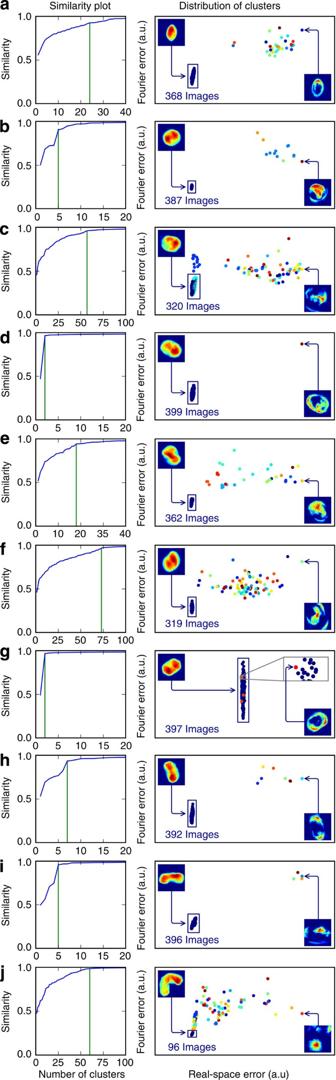Figure 7: Results of clustering. (a–j) The similarity plots with the chosen number of clusters indicated by the vertical line and the scatter plots of the Fourier versus real-space errors for each individual reconstruction (also indicated by (a–j) inFig. 5). Each cluster has been given a unique colour. The image in the top left corner of each scatter plot is an average of all reconstructions in the largest cluster (indicated by the dark blue box). The image in the bottom left corner of each scatter plot is the image of an outlying (or failed) reconstruction. a.u.=arbitrary units. Figure 7: Results of clustering. ( a – j ) The similarity plots with the chosen number of clusters indicated by the vertical line and the scatter plots of the Fourier versus real-space errors for each individual reconstruction (also indicated by ( a – j ) in Fig. 5 ). Each cluster has been given a unique colour. The image in the top left corner of each scatter plot is an average of all reconstructions in the largest cluster (indicated by the dark blue box). The image in the bottom left corner of each scatter plot is the image of an outlying (or failed) reconstruction. a.u.=arbitrary units. 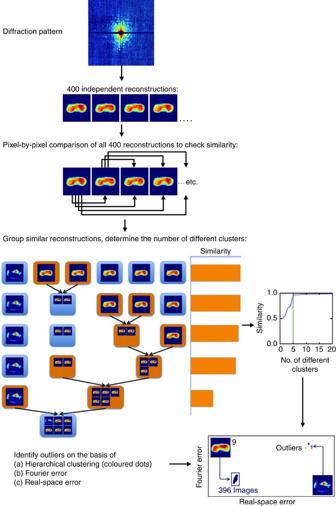Figure 8: Flow chart of image reconstruction. Reconstructions for image 6 fromFig. 5were used in this flow chart. Full size image Figure 8: Flow chart of image reconstruction. Reconstructions for image 6 from Fig. 5 were used in this flow chart. Full size image The results of clustering are shown in Fig. 7a–j . On average about 370 out of 400 reconstructions were considered successful (93%) and kept for further analysis in all cases, except for one case where only 96 reconstructions formed the biggest cluster ( Fig. 7j ). The similarity plots in Fig. 7 show the chosen number of clusters (indicated by the vertical line). The figure also shows the scatter plots of the Fourier errors versus the real-space errors for each reconstructed image from Fig. 5 . The colour of the dots indicates different clusters. The image in the top left corner of each scatter plot is the final, averaged reconstruction of all selected reconstructions in the dark blue box. The image in the bottom right corner of each scatter plot shows an example of an individual reconstruction regarded as an outlier, based on the error measures and/or clustering assignment. Clustering validates the results from using a threshold on the Fourier-error and the real-space error. In most cases, the main cluster has a distinctly lower Fourier-error and real-space error compared with other clusters, making us believe this is the true reconstruction minimum. Reconstructions with higher errors are very different from reconstructions with lower errors, suggesting that failed reconstructions did not reach the true minimum for these reconstructions. The scatter plots of Fig. 7a–j show that the real-space error is more reliable than the Fourier-error for identifying failed reconstructions. Furthermore, clustering aids in the identification of failed reconstructions, as it does for reconstruction 7, even if the error measures are not different. In the case that several large clusters remaining after applying a real-space error and Fourier-error threshold the clusters have to be examined carefully. If the cluster correlates with the errors, we keep the cluster with the lowest error, otherwise we suggest keeping all clusters for further evaluation. In the latter case there is a possibility of over clustering. Figure 8 shows the flow chart of the image reconstruction process. Data deposition statement Data will be deposited with the Coherent X-ray Imaging Data Bank (http://www.cxidb.org). How to cite this article: van der Schot, G. et al . Imaging single cells in a beam of live cyanobacteria with an X-ray laser. Nat. Commun. 6:5704 doi: 10.1038/ncomms6704 (2015).